Active learning framework with iterative clustering for bioimage classification Advances in imaging systems have yielded a flood of images into the research field. A semi-automated facility can reduce the laborious task of classifying this large number of images. Here we report the development of a novel framework, CARTA (Clustering-Aided Rapid Training Agent), applicable to bioimage classification that facilitates annotation and selection of features. CARTA comprises an active learning algorithm combined with a genetic algorithm and self-organizing map. The framework provides an easy and interactive annotation method and accurate classification. The CARTA framework enables classification of subcellular localization, mitotic phases and discrimination of apoptosis in images of plant and human cells with an accuracy level greater than or equal to annotators. CARTA can be applied to classification of magnetic resonance imaging of cancer cells or multicolour time-course images after surgery. Furthermore, CARTA can support development of customized features for classification, high-throughput phenotyping and application of various classification schemes dependent on the user's purpose. Imaging has a vital role in various fields of the life sciences, including cell biology, developmental biology, systems biology and medical sciences [1] . The development of various fluorescent proteins and probes has allowed a wide range of imaging modalities to be used to acquire images of biological structures and specific molecules [2] , [3] . The innovation of high-throughput fluorescence microscopy has quickly led to the acquisition of vast amounts of image data sets by large-scale projects, for example, genome-wide RNA interference (RNAi) screening [4] and location proteomics [5] . Time-lapse confocal microscopy of living cells or organs can be used to monitor the in vivo status of the cells including proliferation, movement and morphological changes based on multidimensional data [4] . Several dedicated imaging systems used in medicine can also render complex data as high-resolution images, including X-ray computed tomography, magnetic resonance (MR) imaging, single-photon-emission computed tomography and positron emission tomography [6] . These advances in imaging have thus resulted in a large number of images available to researchers, and this in turn has led to a need for the application of semi-automated or fully automated image analyses. Classification is a core technique for image analysis. Several methodologies for biological image classification have been developed [1] . The machine learning method has been adapted to image classification and can be broadly divided into two methods, supervised learning and unsupervised learning [7] . As supervised learning methods, nearest neighbour [8] or support vector machine (SVM) [9] are often used to train an image classifier, in which users are required to categorize a part of the image set (training images) into several classes. In this paper, this kind of user involvement is referred to as 'annotation'. As a result of the requirement for user-based training, the constructed classifier often lacks versatility. To classify images for different purposes, the user must re-categorize the training images and re-construct the image classifier, requiring laborious user involvement for bioimage analysis. In contrast, unsupervised learning algorithms do not require categorization information. Although such methods cannot categorize each image into a user-defined class, they can provide important cues for image classification in the form of a two-dimensional plot or dendrogram. The degree of similarity between images can be demonstrated via principal component analysis [10] and multidimensional scaling [11] , both of which are unsupervised learning methods. A user can visually inspect categories of images based on this similarity. However, a problem sometimes arises where clustering includes a category with unrelated biological features such as imaging noise or different intensities in image incorporation. In addition to supervised learning and unsupervised learning, in recent years new kinds of machine learning algorithms have emerged such as semi-supervised learning [12] and active learning [13] . These algorithms were proposed to reduce the cost for annotation and classifier training. In the semi-supervised learning method, the classifier is constructed from unannotated data in addition to annotated data. The type of semi-supervised learning algorithm can be divided into several categories depending on how unannotated data is incorporated into the classification model: self-training [14] , co-training [15] , expectation maximization with a generative mixture model [16] and transductive SVM [17] . On the other hand, the active learning method is an interactive algorithm that picks up part of the unannotated data as a query for the user and increases the amount of annotated data gradually [18] . The active learning method aims to construct an accurate classifier with the least amount of annotation. To generate the rewarding query from unannotated data, several algorithms have been proposed and are in use, including uncertainty sampling [19] , query-by-committee [20] , expected model change [21] , expected error reduction [22] and variance reduction [23] . The semi-supervised learning and active learning methods both try to use an abundance of unannotated data to train an accurate classifier. These approaches have a wide field of application such as in medical image analysis, text classification and voice recognition. However, these approaches are not intended to facilitate the annotation task itself. Improvement of the annotation style during active learning will further reduce the user's task while maintaining the accuracy of the classification. Here we describe a novel active learning framework with interactive clustering for bioimage classification to reduce the human labour cost for annotation and enhance versatility in image classification. In contrast to the existing methods of semi-supervised learning and active learning framework, we focus on the ease of interactive annotation. To accomplish this aim, we developed a visualization method, which is suitable both for browsing of images and for flexible response to the annotation. We call this system CARTA (Clustering-Aided Rapid Training Agent), which is also derived from 'card' in Portuguese and a Japanese card game 'karuta'. CARTA includes a new active learning algorithm that integrates supervised learning methods with an unsupervised learning algorithm, the self-organizing map (SOM). A SOM can perform nonlinear projections of high-dimensional data onto a two-dimensional map with preservation of high-dimensional topology, facilitating visualization and interpretation of clustering results [24] , [25] , [26] . Moreover, a SOM is more robust to data with outliers or without a normal distribution and can maximize data visualization over the area of the computer monitor. SOMs have been adapted to various analyses of massive data sets including genome informatics [27] and gene expression analysis [28] , [29] . CARTA is a potentially useful framework for incorporating SOMs into bioimage classification to supply a universal platform for a wide range of imaging systems. A SOM has the advantage of being able to browse the images. In CARTA, the user can easily inspect image categories by SOM visualization on the computer monitor. CARTA also has the ability for data mining. A SOM enables unexpected categories to be found by the survey of image distribution through effective visualization. Framework of CARTA To speed up the annotation task with minimal effort, CARTA provides an interactive interface for displaying unannotated images to the user in an organized manner. Suppose, given a set of N input images, D features are extracted from each image, where N is the total number of input images and D is the total number of features. Each image then appears as a point x in the feature space R D . It is a feature vector x composed of D component values in the D -dimensional coordinates. Input images can be described by a set of N vectors such that X ={ x 1 , x 2 , ... x N }, x ∈ R D . As with active learning, the user adds annotation information y to image x as to which class the image x belongs to. Let y i ={0} ∪ {1, 2, ... K } denote the labels of image x i , where 0 represents 'unannotated' and K is the total number of classes, and the annotation status of image set X is represented by Y ={ y 1 , y 2 , ... y N }. To facilitate the user-driven annotation task, the distribution of image set X in the high-dimensional feature space R D should be visualized in an ordered manner on the two-dimensional coordinate system. At the same time, as the total number of images N is too large to be displayed simultaneously, some representative images should be selected and assigned onto the two-dimensional rectangular grid. Each of the images are parameterized with respect to an integer coordinate pair Q 1 × Q 2 . Here Q 1 ={1, 2, ..., q 1 }, and similarly for Q 2 . Let f ( x ) denote the position of grid Q 1 × Q 2 , the function f maps the feature space to the grid: In contrast to the conventional active learning approach, CARTA aims to achieve a further efficiency by allowing the user to select unannotated images for annotation from the representative images ordered by some sort of criteria on the rectangular grid Q 1 × Q 2 . The reason for this is that the annotation task by a comparison of ordered images is easier and faster than the individual and repeated annotation of each image, even for experts. As a result of the annotation, the labels of the input images Y are updated. Because the function f is for the display to the user and the optimal form of f is dependent on the properties of the input images and the user's intent, we cannot obtain the optimal f in advance. The properties of the images are represented by feature vectors X through feature extraction. The user's intent for classification is represented by the annotation status Y , which is dynamically updated by active learning. Then we can estimate function f for the specific images and each intent using X and Y . Let a function V be the evaluation function of f , then the optimization of f can be formulated as Because the function V has the argument Y , which can vary with every cycle of the annotation, CARTA searches for the suboptimal f asymptotically and synchronously to the annotation step. Implementation of CARTA framework To implement the CARTA framework, we aimed to combine simple methods in an effort to achieve general versatility and simplicity. In that context, the function f is composed of a feature-selecting function g and SOM function h . At first, function g selects some features from the feature vector x ∈ R D , therefore, an input image is mapped to a vector in lower dimensional feature space as g ( x ) ∈ R S , where S is a number of selected features and D ≥ S ≥ 1. Next, function h tiles the images on the rectangular grid Q 1 × Q 2 . Taken together, formula (1) is performed by functions h and g via the subspace R S : Then we focus on the optimization of function g , which compresses the input image onto the feature subspace R S : Function g can be perceived as a feature filter that select S features from D features, and in that respect CARTA can also be used as a solving tool for feature-selection problems (FSPs) [30] . We used the genetic algorithm (GA) as an optimization technique for finding the suboptimal solution from multiple candidates: 2 D −1 combinations. The GA, which imitates biological reproduction and natural selection [31] , has the advantages that it is free from the need for parameter tuning and it converges quickly. Because of this, the GA has already been used in FSP solver [32] . We define the function V , which is the target of optimization, as following: where d k is the intra-class distance of class k on the rectangular grid Q 1 × Q 2 . As the intra-class distance, CARTA use the sum of edge length in minimum-spanning tree (MST) [33] on the grid. From a different viewpoint, the flow of CARTA until the construction of the classifier is as follows. Initially, CARTA extracts all features from the images using the feature extractor ( Fig. 1a ). The features can be referred to as Kashiwa bioimaging (KBI) features ( http://hasezawa.ib.k.u-tokyo.ac.jp/zp/Kbi/KbiFeatures02 ). The KBI feature extractor internally performs three thresholding algorithms including Otsu's method [34] and image correlation spectroscopy [35] ( Fig. 1b ). Based on randomly selected features, the SOM viewer in CARTA displays an 'initial SOM' to show the distribution of images with representative images, which are displayed from an image group in the same node. The user can then easily categorize the represented images by delineating lines on the initial SOM as highlighted by blue in Fig. 1a , a process referred to as annotation in this paper. The annotation information is then incorporated into the feature optimizer (FO). The FO selects appropriate features to segregate images into different classes by GA. The SOM generator then prepares an 'updated SOM' from the selected features. The selected features are also displayed to the user by showing allocated numbers. The feature evaluator then evaluates the validity (the function V in equation (3)) of the SOM clustering as the distance between the images that are annotated as the same groups in the SOM. The evaluated results are incorporated into the FO. The FO selects features again based on the evaluated results. The user can again annotate the represented images by the updated SOM ( Fig. 1a ). The iterative process can be stopped at any time according to the user's judgment by monitoring the fitness curve of the function V , or it can be automatically stopped in the event that the fitness does not improve within a user-defined generation interval in the GA ( Fig. 1c ). After clustering at the end of CARTA, selected features are transferred into the classifier generator using SVM. Once the classifier is trained, newly supplied images can be automatically classified into the user-defined categories with the classifier. 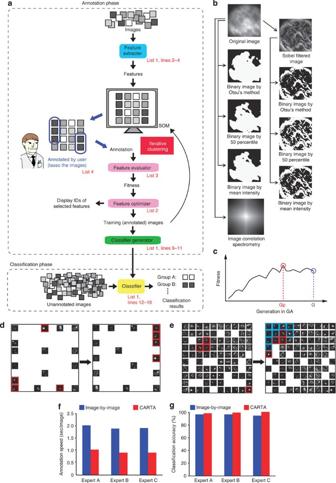Figure 1: Bioimage clustering and classification by CARTA. (a) Workflow of CARTA algorithm that is composed of the annotation and classification phase. Lists and lines in red correspond to the pseudocode as shown inSupplementary Software 1. (b) Pipeline of image processing for extraction of KBI features. (c) Example for a fitness curve in the iterative clustering with generations in genetic algorithm (GA). Gp and G shows peakGeneration and generation as shown in List 2 ofSupplementary Software 1, respectively. (d) Upgrade of the self-organizing map (SOM) in CARTA. The initial SOM shows the arrangement of 16 fluorescent images of green fluorescent protein (GFP) localization (GFP-AtORF database)36(left panel). After the annotation of images to show nuclear localization in the red open boxes, the updated SOM shows the gathering of annotated images in the right upper region (right panel). (e) Identification of unannotated images by CARTA. The initial SOM shows the arrangement of 155 fluorescent images of GFP localization (GFP-AtORF database)36with 83 representative images (left panel). After the annotation, the updated SOM shows the grouping of annotated images in red open boxes and unannotated images in blue boxes in the left upper region (right panel). (f,g) Comparison of annotation speed (f) and accuracy (g) between image-by-image annotation and annotation with CARTA. We prepared 82 images of prophase/prometaphase chromosomes within HeLa cells. Three expert observers annotated the image set image-by-image or by using CARTA. Figure 1: Bioimage clustering and classification by CARTA. ( a ) Workflow of CARTA algorithm that is composed of the annotation and classification phase. Lists and lines in red correspond to the pseudocode as shown in Supplementary Software 1 . ( b ) Pipeline of image processing for extraction of KBI features. ( c ) Example for a fitness curve in the iterative clustering with generations in genetic algorithm (GA). Gp and G shows peakGeneration and generation as shown in List 2 of Supplementary Software 1 , respectively. ( d ) Upgrade of the self-organizing map (SOM) in CARTA. The initial SOM shows the arrangement of 16 fluorescent images of green fluorescent protein (GFP) localization (GFP-AtORF database) [36] (left panel). After the annotation of images to show nuclear localization in the red open boxes, the updated SOM shows the gathering of annotated images in the right upper region (right panel). ( e ) Identification of unannotated images by CARTA. The initial SOM shows the arrangement of 155 fluorescent images of GFP localization (GFP-AtORF database) [36] with 83 representative images (left panel). After the annotation, the updated SOM shows the grouping of annotated images in red open boxes and unannotated images in blue boxes in the left upper region (right panel). ( f , g ) Comparison of annotation speed ( f ) and accuracy ( g ) between image-by-image annotation and annotation with CARTA. We prepared 82 images of prophase/prometaphase chromosomes within HeLa cells. Three expert observers annotated the image set image-by-image or by using CARTA. Full size image To validate the classification ability of CARTA, we tried to identify images with a specific subcellular localization pattern in the green fluorescent protein (GFP) database (GFP-AtORF DB; http://data.jic.bbsrc.ac.uk/cgi-bin/gfp/ ) in plants [36] . Improvement of SOM clustering was clearly shown by gathering the distribution of four images that the user annotated to show single nuclei (right upper region) from the randomly selected 16 images ( Fig. 1d ). CARTA was also useful for identifying unannotated images with specific GFP localization from the image database. All images (155 images) from the database were applied to CARTA ( Fig. 1e ). CARTA was able to gather images that were annotated by the user and at the same time, unannotated images with nuclear localization located around the annotated images. This result demonstrates that CARTA can identify analogous images from a large image database using only the annotation of a few images. Moreover, based on subcellular localization of GFP signals, the 155 images in the GFP-AtORF database were classified into five classes, including 'cytoplasm', 'nuclear', 'nucleolar', 'cell wall' and 'others', in the database. For the classification of 'cytoplasm', 'nuclear' and 'cell wall', CARTA performed better than human annotators who were experts in studying plant cell biology ( Table 1 ). Table 1 Comparison of subcellular localization of GFP-fused proteins in plant-cultured cells. Full size table To demonstrate the efficiency of using CARTA to perform annotation, we measured the time required for three experts to annotate the fluorescence images. CARTA was successful in decreasing the annotation time to 49% of that of image-by-image annotation ( Fig. 1f ) while maintaining the same level of accuracy ( Fig. 1g ). Efficient browsing in CARTA The SOM, which is also called a 'tiled' map in this study, is an excellent browser for exhibiting the image group as a node in a lattice map. The representative images, which are selected from the majority of images at each node, are positioned ( Fig. 2a ). However, if a large amount of images are arranged on the SOM, each node includes many images and the user has no way of revealing the proportion of different types of images at the node. To visualize the proportions of image types in the node, CARTA can produce a pie chart map in addition to a tiled map. In the pie chart map, the colour sectors demonstrate the proportion of image types and the size of the circle is proportional to the number of images at each node ( Fig. 2b ). The pie chart map can summarize the annotated images and illustrate the image type proportion in each node. 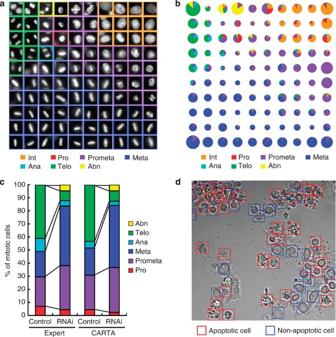Figure 2: Automatic classification of mitotic phases by CARTA. A tiled map (a) and a pie chart map (b) of 4,598 fluorescent images of the dynamics of nuclei and chromosomes in human cultured cells. The frames of representative images and colour sectors of the pie chart indicate the class of mitotic phases including interphase (Int) in orange, prophase (Pro) in red, prometaphase (Prometa) in purple, metaphase (Meta) in blue, anaphase (Ana) in light blue and telophase (Telo) in light green. Abnormal cells (Abn) in yellow include apoptotic cells. The pie chart size is proportional to the number of images at the node. (c) Comparison of classification of RNAi cells by a human annotator and CARTA. (d) Discrimination of apoptotic cells in a differential interference contrast image using a CARTA classifier. Differential interference contrast images of apoptosis-induced HeLa cells were classified by CARTA. The red and blue windows show apoptotic and non-apoptotic cells, respectively. Figure 2: Automatic classification of mitotic phases by CARTA. A tiled map ( a ) and a pie chart map ( b ) of 4,598 fluorescent images of the dynamics of nuclei and chromosomes in human cultured cells. The frames of representative images and colour sectors of the pie chart indicate the class of mitotic phases including interphase (Int) in orange, prophase (Pro) in red, prometaphase (Prometa) in purple, metaphase (Meta) in blue, anaphase (Ana) in light blue and telophase (Telo) in light green. Abnormal cells (Abn) in yellow include apoptotic cells. The pie chart size is proportional to the number of images at the node. ( c ) Comparison of classification of RNAi cells by a human annotator and CARTA. ( d ) Discrimination of apoptotic cells in a differential interference contrast image using a CARTA classifier. Differential interference contrast images of apoptosis-induced HeLa cells were classified by CARTA. The red and blue windows show apoptotic and non-apoptotic cells, respectively. Full size image Accurate classification by CARTA To evaluate the accuracy of CARTA, we used fluorescent images of HeLa cells expressing histone H1 fused with GFP [37] in the control and ASURA (PHB2) RNAi experiments. ASURA-knockdown induces mitotic delay [38] . A mixture of 4,598 images were manually classified into seven classes based on nuclei or chromosome morphology: interphase, prophase, prometaphase, metaphase, anaphase, telophase, and abnormal phenotypes including apoptosis. Using the image features and these annotations, we finally obtained the classifier by the SVM using 186 features. The classification accuracy reached ∼ 90% ( Fig. 2c ) as visualized by the SOM ( Fig. 2a,b ). The accuracy was maintained at a high level when the class number increased by class separation ( Fig. 2c ). The output of the classifier showed the same percentage of mitotic phases in the control and RNAi cells as that with classification by an expert ( Fig. 2c ) [38] . This result shows that discrimination of mitotic phases by an expert can be replaced by CARTA. CARTA can also classify several types of images other than fluorescent images, as well as feedback the classification results to the original images. Using the classifier based on annotation of differential interference contrast images of 300 apoptotic cells, CARTA can morphologically discriminate apoptotic cells from differential interference contrast images without apoptotic indicators with 98.4% accuracy as compared with researchers ( Fig. 2d ). We evaluated the performance of CARTA as compared with commercial software, the Cell Cycle application module in version 7.5 Metamorph (CCAM) software. The accuracy of CCAM with the same image sets used with CARTA was reduced below 70% mainly because CCAM treated a cluster of chromatids as two different nuclei or chromatids ( Fig. 3a,b ). In addition, CCAM was not robust to the GFP expression level, because it depends on the absolute values of the intensity. This demonstrates the limitation of the built-in features used in CCAM. 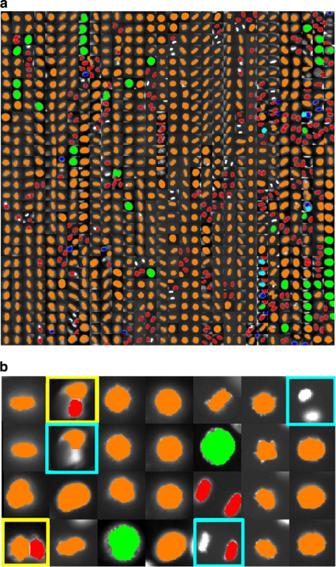Figure 3: Classification of mitotic phases by a commercially available software. (a) A tiled map of the same 900 images classified by the application module in the Metamorph software. The images are same as those classified by CARTA inFig. 2. Blue, green, orange and red indicate cells in interphase at G1/S phase, interphase nuclei at G2 phase, in early M phase and in late M phase, respectively. (b) A magnified area of the tiled map. The yellow box shows an erroneous classified image where the application module treated a cluster of chromatids as two different nuclei or chromatids. The light blue box shows another erroneously classified image where the application module could not classify images over the assigned intensity. Figure 3: Classification of mitotic phases by a commercially available software. ( a ) A tiled map of the same 900 images classified by the application module in the Metamorph software. The images are same as those classified by CARTA in Fig. 2 . Blue, green, orange and red indicate cells in interphase at G1/S phase, interphase nuclei at G2 phase, in early M phase and in late M phase, respectively. ( b ) A magnified area of the tiled map. The yellow box shows an erroneous classified image where the application module treated a cluster of chromatids as two different nuclei or chromatids. The light blue box shows another erroneously classified image where the application module could not classify images over the assigned intensity. Full size image Semi-automatic classification of biomedical images using CARTA Irregular and complex medical images create difficulties for accurate clinical examination. One of most important diagnostic tasks in cancer imaging is the identification of the origin of tumours, which contributes to the selection or determination of therapy [39] . Pathological diagnosis is the gold standard method. However, in many cases, biopsy for pathological diagnosis cannot be performed due to the potential for complications [40] . In contrast, the identification of the origin of tumours by diagnostic imaging depends on the proficiency of the medical specialist. Thus, to test the feasibility of using CARTA for the automatic identification of the origin of tumours, we used MR images of tumours that were induced by subcutaneous injection of different cancer cells. S180 and FM3A, which are derived from sarcoma and mammary cancers, respectively, were transplanted into mice. Two hundred sixty-eight images were collected from tumours on 19 individual mice. CARTA separated the tumour images derived from S180 and FM3A in the lower and upper regions in the SOM ( Fig. 4a,b ), and achieved 94.0% classification accuracy. Such accurate classification of MR images by CARTA demonstrates the potential for automatic discrimination of tumour cell origins. 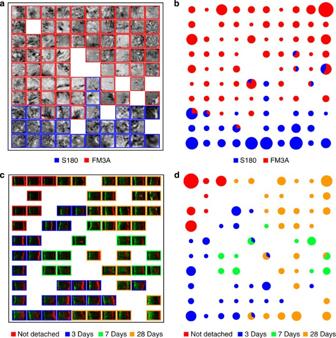Figure 4: Automatic classification of biomedical images. A tiled map (a) and a pie chart map (b) of magnetic resonance images of mouse tumours. Two hundred sixty-eight images of tumour were classified by CARTA. Blue and red frames show representative images corresponding to S180 and FM3A cancer cells, respectively. A tiled map (c) and a pie chart map (d) of colour images of detached cat retinas. One hundred seventy-one images of rod photoreceptors and microglia in cat retinas were visualized by anti-rod opsin antibody in red and anti-isolectin B4 antibody in green. Representative images of no detachment and 3, 7 and 28 days after detachment are shown in the red, blue, green and orange frames, respectively. Figure 4: Automatic classification of biomedical images. A tiled map ( a ) and a pie chart map ( b ) of magnetic resonance images of mouse tumours. Two hundred sixty-eight images of tumour were classified by CARTA. Blue and red frames show representative images corresponding to S180 and FM3A cancer cells, respectively. A tiled map ( c ) and a pie chart map ( d ) of colour images of detached cat retinas. One hundred seventy-one images of rod photoreceptors and microglia in cat retinas were visualized by anti-rod opsin antibody in red and anti-isolectin B4 antibody in green. Representative images of no detachment and 3, 7 and 28 days after detachment are shown in the red, blue, green and orange frames, respectively. Full size image To confirm the ability of CARTA for evaluation of colour tissue images, we classified images of retinal layers within the UCSB benchmark data set ( http://www.bioimage.ucsb.edu/biosegmentation/ ). Evaluation of structural and cellular changes in the retina is a crucial step in the examination of injury and disease. One hundred seventy-one confocal microscopic images of detached cat retinas were classified. CARTA was able to accurately classify these features according to retina recovery after detachment ( Fig. 4c,d ). The specific distribution of image groups included images of 'no detachment', '3 days after detachment (d.a.d. )', '7 d.a.d.' and '28 d.a.d.' These data indicate that CARTA can automatically classify biomedical images into appropriate categories for clinical judgment, demonstrating that CARTA has the ability to reduce the effort required of medical specialists to classify images. Use of customized features for image classification CARTA can use user-defined features for image classification. Therefore, users can replace the KBI features with more appropriate features according to the desired classification purpose. To demonstrate this advantage of CARTA, we compared the KBI features and threshold adjacency statistics (TAS) features that were previously used for fluorescence-tagged protein localization with iCluster software [41] . Nocodazole-treated and untreated images of the endosomal protein SNX1 are freely available in http://icluster.imb.uq.edu.au/imagesets.html , and were classified as a benchmark test. The accuracy was 98.1% and 96.9% with KBI and TAS features ( Fig. 5a ), respectively, suggesting that KBI features are comparable to TAS features in fluorescence protein localization analysis. To test for the differences of these features, we added Gaussian noise to the original images. TAS features achieved higher accuracy when the noise was magnified ( Fig. 5a ). These results indicated that KBI features are acceptable for the initial analysis choice. If users are unsatisfied with the results obtained with the KBI features, they can freely replace them with the alternative features like TAS features as customized features. 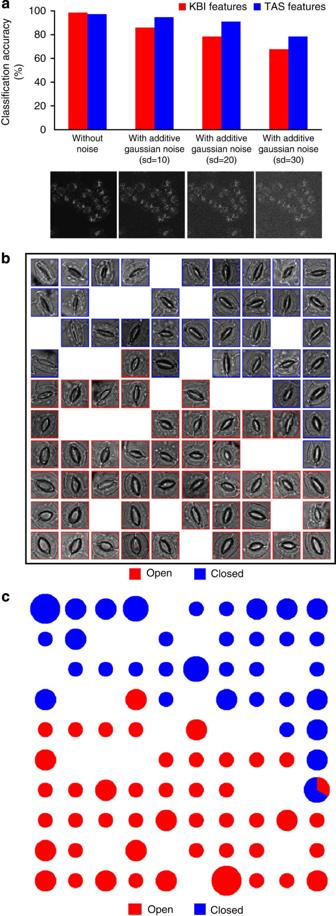Figure 5: Exploitation of customized features in CARTA. (a) Comparison of classification accuracy between KBI features and threshold adjacency statistics (TAS) features. Qualities of fluorescent images are artificially reduced by additive white Gaussian noise. (b) A tiled map of stomata in the leaves ofArabidopsis thaliana. Representative images of open and closed stomata are shown in red and blue open boxes. (c) A pie chart map of open and closed stomata. Red and blue sectors of the pie charts demonstrate the proportion of images of open and closed stomata at the node. The size of the pie chart is proportional to the number of images. Figure 5: Exploitation of customized features in CARTA. ( a ) Comparison of classification accuracy between KBI features and threshold adjacency statistics (TAS) features. Qualities of fluorescent images are artificially reduced by additive white Gaussian noise. ( b ) A tiled map of stomata in the leaves of Arabidopsis thaliana . Representative images of open and closed stomata are shown in red and blue open boxes. ( c ) A pie chart map of open and closed stomata. Red and blue sectors of the pie charts demonstrate the proportion of images of open and closed stomata at the node. The size of the pie chart is proportional to the number of images. Full size image We encountered a difficult problem in the classification of opened/closed stomata, a pore for gas and water exchange of plants. When the combination of features to discriminate between open and closed conditions of stomata was searched by CARTA, KBI features were insufficient because they were affected by the direction of stomata. Thus, we introduced new rotation-invariant features based on the statistics of intensity on concentric circle (see Supplementary Methods for a definition). By use of 130 rotation-invariant features, CARTA distinctly separated 114 images into different SOM regions consisting of open or closed stomata ( Fig. 5b,c ). This result demonstrates that CARTA can improve classification performance by the introduction of user-customized features. CARTA is a novel algorithm that combines active learning and interactive annotation based on the distribution of input images. Such a combination focuses on the reduction of human labour costs in contrast to supervised learning alone, which consumes longer time [42] . In the active learning paradigm, a classification model is at first temporarily generated from annotated samples by some supervised learning algorithm. By using the classification model, the active learner selects an ambiguous sample that is least certain how to label from the pool or stream of unannotated samples. For example, when using a probabilistic model for binary classification, the active learner queries the sample whose posterior probability of being positive is nearest to 0.5 (refs 43 , 44 ). Thus, the active learning empirically reduces the number of annotations required to achieve a given level of accuracy [45] . In addition, several theoretical analyses have reported that certain active learner strategies require fewer annotations to achieve the same error as the standard supervised algorithm [46] , [47] . For simplicity, we consider the simple example where the unannotated samples can be mapped onto the one-dimensional feature space, and can be split by some threshold into two categories. In that case, a standard supervised learning acts similar to a random search algorithm and requires O (1/ ɛ ) annotations, where ɛ is the maximum desired error rate. On the other hand, an active learner including CARTA acts like a binary search algorithm and requires only O (log 1/ ɛ ) annotations [18] . Furthermore, CARTA takes a set of unannotated images as input and presents to the user the part of images as query for annotation. From this aspect, CARTA can be considered an improved type of batch-mode active learning [48] . The batch-mode active learning is an extended algorithm of active learning to increase the number of query samples per iteration. When compared with batch-mode active learning, CARTA allows the user to decide whether and what images should be annotated, and represents the image sets by similarity-based order to assist the user's decision using SOM. CARTA uses the SOM not only to visualize the images but also to help with annotation. Previous methods have used static clustering including SOMs as only a browser of clustering results to show the data distribution [25] , [26] , [27] , [28] , [29] . In contrast, the SOMs in CARTA can be repeatedly trained and optimized by GA [31] . The update of the SOM contributes to the minimum annotation, meaning that CARTA avoids the laborious annotation of numerous images. In fact, CARTA could halve the annotation time while maintaining classification accuracy ( Fig. 1f,g ). Such similarity-based visualization has attracted attention for the purpose of reducing a user's cognitive effort in content-based image retrieval [49] . For example, tree-structured SOM had been extended to organize the images on the World Wide Web and adapt to the user's preferences in selecting which images resemble each other [50] . Therefore, to our knowledge, CARTA is the first algorithm of an active learning framework that uses the tiled and ordered set of images for bioimage classification. The CARTA algorithm can be used for bioimage classification by a wide range of methods with acceptable accuracy in different image databases ( Fig. 5a ) and images acquired by various imaging systems ( Figs 2 , 4 and 5 ). Moreover, CARTA can allow human experts to evaluate existing feature sets ( Fig. 5a ) and develop novel features ( Fig. 5b,c ). In the computer vision community, a large number of feature libraries have been and will continue to be developed. Among them, the algorithm of CARTA especially fits global image features such as colour histograms, grey-level of co-occurrence matrix [51] and gist descriptor [52] , [53] . The adaptivity for different feature sets will expand the application range of CARTA. Automatic or semi-automatic classification frameworks such as CARTA can enable not only high-throughput but also innovative phenotyping. Algorithm of CARTA The algorithm is given in Supplementary Software 1 and 2 as pseudocode. A flowchart of Supplementary Software 1 is shown in Fig. 1a . CARTA takes as an input a set of images and extracts feature vectors from each image ( Supplementary Software 1 List 1 lines 2–4). From the input images and feature vectors, iterative clustering ( Supplementary Software 1 List 1 line 6, function iterativeClustering in Supplementary Software 1 List 2) simultaneously performs the solving of the FSP and interactive annotation as described in detail below. The selected features are displayed to the user ( Supplementary Software 1 List 1 line 7) and the classification accuracy is estimated by the cross-validation test ( Supplementary Software 1 List 1 lines 9 and 10, function trainAndValidate in Supplementary Software 2 List 7). CARTA does not directly train the final classifier from selected features in contrast to many FSP algorithms. Because modern supervised learning algorithms such as SVM are robust to irrelevant features, the preceding feature selection step sometimes limits the accuracy. Therefore, CARTA compares the classification accuracy obtained from the cross-validation test to determine whether the classifier using a selected feature set is better than that achieved using all features ( Supplementary Software 1 List 1 lines 9–12). Finally, all images including the unannotated images are classified by the improved classifier ( Supplementary Software 1 List 1 lines 12–15, function classify in Supplementary Software 2 List 8). CARTA uses an iterative clustering ( Supplementary Software 1 List 2) for optimizing and annotating step using an interactive GA combined with SOM. GA has previously been used to solve FSP by searching for the combination of useful features in supervised learning [54] , [55] , [56] . In CARTA, each individual chromosome in the GA population represents selected features as in the previous reports, namely, a chromosome is the vector, which is zero or one in each component and its dimension is equal to the feature vector. Initially, S features ( S is smaller than or equal to the dimension of feature vector D ) are randomly selected and are assigned to each individual in the first population ( Supplementary Software 1 List 2 line 8, procedure makeFirstGeneration in Supplementary Software 2 List 5). To speed up the convergence of the optimization, CARTA adopts the m-feature operators, which limit the number of selected features [32] ( Supplementary Software 2 List 5 line 12). Subsequently, the main loop of GA ( Supplementary Software 1 List 2 lines 10–38) is performed to evolve a better set of features. CARTA then evaluates the fitness value of each individual according to the result of SOM ( Supplementary Software 1 List 2 line 12, procedure evaluate in Supplementary Software 1 List 3), to be described later. In CARTA, the generation that achieved the best-fitness value (peakGeneration in Supplementary Software 1 List 2) is used to stop the main loop ( Supplementary Software 1 List 2 line 21) and is updated using a record of the fitness value of each generation ( Supplementary Software 1 List 2 lines 14–37, Fig. 1c ). In addition, the user can stop the loop when the best-fitness value becomes saturated ( Supplementary Software 1 List 2 line 21) by monitoring the history of the fitness values ( Supplementary Software 1 List 2 line 16). As the interactive GA, CARTA accepts user annotation during the main loop of GA ( Supplementary Software 1 List 2 line 24, function acceptAnnotation in Supplementary Software 1 List 4). Using the best-selected features (peakSelector in Supplementary Software 1 List 2), the SOM is trained in the feature subspace ( Supplementary Software 1 List 4 lines 2–3) and all images are dispatched into their best-matching units in the SOM ( Supplementary Software 1 List 4 lines 4–7). Next, for each node of SOM, one image is selected from the dispatched images into the node and displayed to the user ( Supplementary Software 1 List 4 lines 8–12). The user can recognize the distribution of input images by monitoring only the representative image of each node ( Fig. 1d,e ). Optionally, the user can annotate the displayed images by tagging the class label that the image should be classified with ( Supplementary Software 1 List 4 lines 13–14). When the user annotates some images, the best-fitness value is discarded ( Supplementary Software 1 List 2 line 26), as the criteria for fitness will have changed. All annotated information is accumulated ( Supplementary Software 1 List 2 lines 29–34) and is applied to the next evaluation step ( Supplementary Software 1 List 2 lines 11–13) and the training of classifiers ( Supplementary Software 1 List 1 lines 9–10). The generation change of CARTA ( Supplementary Software 1 List 2 lines 36–37) is described in Supplementary Software 2 List 6 (function makeOffsprings). It adopts a tournament selection, a uniform crossover and point mutation ( Supplementary Software 2 List 6 lines 7–10). After the mutation step, m-feature operators are additionally applied to limit the number of selected features [32] ( Supplementary Software 2 List 6 line 11) to the same as the initial population ( Supplementary Software 2 List 5 line 12). From the point of view of the fitness evaluation ( Supplementary Software 1 List 2 lines 11–13, procedure evaluate in Supplementary Software 1 List 3), the application of GA in the FSP can be divided into two major categories: filter methods and wrapper methods [32] . The filter methods use an indirect measure of the quality of the selected features, so a faster convergence of the algorithm is obtained. On the other hand, wrapper methods use as selection criteria the output of the learning machine. CARTA adopts the filter methods because the supervised-learning machine is unable to train from the input data set of CARTA, unsupervised images. As a measure of the quality of the selected features, the compactness of the SOM of images that are labelled with same class is evaluated. First, CARTA trains a SOM based on all feature vectors projected to subspace according to the selected features ( Supplementary Software 1 List 3 lines 5–6). Second, each class is dispatched to the points on the two-dimensional space by finding the best-matching units of their vectors ( Supplementary Software 1 List 3 lines 8–12). Better features will provide a more compact distribution of the points ( Fig. 1d,e ). Third, CARTA constructs a MST binding all points with minimum links ( Supplementary Software 1 List 3 line 14). The total length of the arcs of MST ( Supplementary Software 1 List 3 line 15) is treated as a raw fitness value indicating the compactness of the points. The raw fitness values for each class are summed to yield the fitness value considering all classes. Finally, the fitness values are adjusted based on the occupancy of all input feature vectors on the SOM ( Supplementary Software 1 List 3 lines 18–22). CARTA construction and performance We have developed a CARTA plugin for ImageJ software [57] (National Institutes of Health, Bethesda, Maryland, USA; http://rsb.info.nih.gov/ij/ ). The CARTA plugin was implemented in the Scala language ( http://www.scala-lang.org/ ) and is executable under Windows, Mac OS X and Linux. Annotations on SOM can be performed using the Freehand selection tool of ImageJ. SVM (libsvm, http://www.csie.ntu.edu.tw/~cjlin/libsvm/ ) [58] was used for supervised learning in CARTA. The libsvm library is automatically called from the CARTA plugin. We used KBI features version 2 that contains 296 features ( http://hasezawa.ib.k.u-tokyo.ac.jp/zp/Kbi/KbiFeatures02 ), but more preferred features can be used for specific purposes as shown in Fig. 5 . The computation takes 0.29 s per image (130×130 pixels) for feature extraction, 8.25 s per generation in GA ( N =64, 20 images, 10×10 SOM) for feature selection, 0.05 s per image for supervised learning, and 0.02 s for classification of new images. Computation was performed on a computer workstation with a Core i7 1.2 GHz processor and 4 GiB of memory. Live cell imaging of RNAi of HeLa cells and apoptotic induction We acquired fluorescent and differential interference contrast images with an automated epifluorescence microscope (IX-81; Olympus, Tokyo, Japan) under a ×40 objective lens with a cooled charged couple detector camera head system (CoolSNAP HQ2; PhotoMetrics, Arizona, USA) using Metamorph software version 7.5 (Molecular Devices, Sunnyvale, California, USA). We incubated HeLa cells onto 35 mm glass-bottomed dishes (Matsunami, Osaka, Japan) and maintained them in DMEM without phenol-red (Invitrogen, California, USA) with 10 mM HEPES (pH 7.2) at 37 °C in a microscopic CO 2 incubator (MI-IBC; Olympus, Tokyo, Japan). RNAi for ASURA (PHB2) was performed as described elsewhere [37] . Induction of apoptosis in HeLa cells was performed by addition of bisphenol A at the final concentration of 10 μM [59] . How to cite this article: Kutsuna, N. et al . Active learning framework with iterative clustering for bioimage classification. Nat. Commun. 3:1032 doi: 10.1038/ncomms2030 (2012).